Phantom pain is associated with preserved structure and function in the former hand area Phantom pain after arm amputation is widely believed to arise from maladaptive cortical reorganization, triggered by loss of sensory input. We instead propose that chronic phantom pain experience drives plasticity by maintaining local cortical representations and disrupting inter-regional connectivity. Here we show that, while loss of sensory input is generally characterized by structural and functional degeneration in the deprived sensorimotor cortex, the experience of persistent pain is associated with preserved structure and functional organization in the former hand area. Furthermore, consistent with the isolated nature of phantom experience, phantom pain is associated with reduced inter-regional functional connectivity in the primary sensorimotor cortex. We therefore propose that contrary to the maladaptive model, cortical plasticity associated with phantom pain is driven by powerful and long-lasting subjective sensory experience, such as triggered by nociceptive or top–down inputs. Our results prompt a revisiting of the link between phantom pain and brain organization. Following arm amputation, individuals often perceive pain in their missing limb. The cause of phantom pain experience has commonly been attributed to maladaptive plasticity: following loss of sensory input, the deprived hand area of the primary sensorimotor cortex becomes responsive to inputs from cortical neighbours (for example, face), thereby triggering pain representations relating to the hand [1] . Over the years, the maladaptive plasticity model has been extended to explain other disorders of pain, motor control and tinnitus [2] , [3] . Moreover, it has inspired rehabilitation strategies aimed at reversing supposed maladaptive plasticity, thus relieving phantom pain [1] , [2] , [4] . The maladaptive plasticity model is most clearly supported by expansions or shifts in cortical lip representations towards the deprived hand area: the greater the remapping, the more severe the pain [5] . Although representations of the missing limb are directly investigated less frequently, the maladaptive plasticity model would predict that such representations should be reduced in the sensorimotor cortex of people who suffer from more pain, owing to greater remapping. Several lines of evidence call this prediction to question. First, volitional non-painful movement of a phantom elicits central [6] and peripheral [7] motor execution signals, suggesting preserved representation. Such signals were not elicited when amputees were instructed to simply imagine moving their phantom limb, similar to dissociations found between actual and imagined movement of an intact limb. Second, phantom sensations, and pain in particular, can be triggered by bottom–up aberrant inputs, such as those relating to peripheral nerve injury [8] . Increased peripheral inputs, associated with phantom pain, might therefore contribute to maintained cortical representation. We propose that over the long term, maintained representation and continued inputs could preserve local cortical structure and function in an experience-dependent manner, such that greater chronic phantom sensation is associated with greater phantom representation. A persistent representation model will therefore predict that phantom pain correlates more strongly with maintained phantom representations, than with shifted lips representation. Moreover, as phantom pain experiences are decoupled from other sensorimotor experiences, the lack of co-activation of the cortical phantom area and other body parts (such as the intact hand) may result in diminished interactions between different body part representations. To revisit the maladaptive plasticity model, we studied the cortical correlates of phantom pain in the area representing the missing hand itself, rather than the representations of the neighbouring (intact) body parts. Using an array of neuroimaging techniques, we discovered that subjective reports of chronic phantom pain experience accounted for much of the variability found between individuals within the phantom cortex: greater phantom pain was associated with more local activity and more structural integrity within the phantom cortex. Phantom pain magnitude was also associated with disrupted inter-regional functional connectivity of the primary sensorimotor cortex at rest. We believe that our findings are best understood in terms of experience-dependent plasticity, with chronic phantom pain providing the experience. 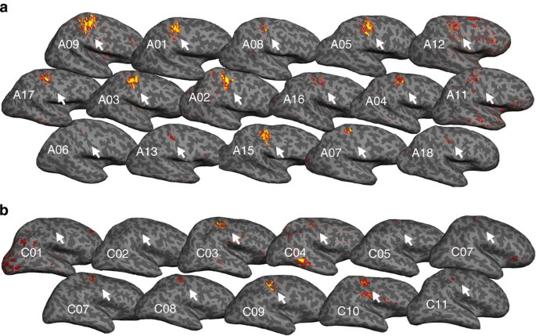Figure 1: Individuals’ missing-hand representations. Activation for movement of phantom hand versus toes in amputees (a) and for imagined missing-hand movements versus toes in 1-handed controls (b), projected on individuals’ inflated contralateral hemisphere. Arrows indicate the position of the central sulcus. Amputees are ordered according to their phantom pain ratings (amputees with greater chronic pain are presented first). Participants’ codes (A01, C01 and so on) correspond toTables 1and2. 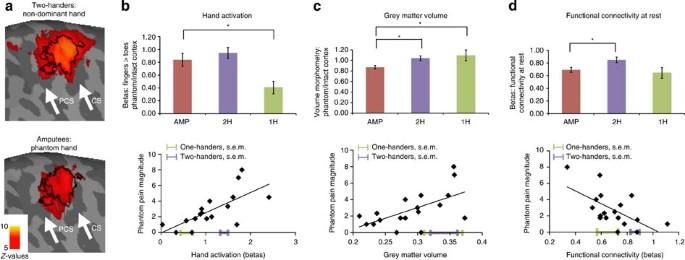Figure 2: Chronic phantom pain relates to maintained local cortical representations and disrupted inter-regional connectivity. (a) Activation for movement of non-dominant and phantom hands versus toes in 2-handed controls (top) and amputees (bottom), projected on an inflated contralateral hemisphere. PCS, postcentral sulcus; CS, central sulcus. Black line delineates the boundaries of the ‘phantom cortex’ ROI. (b–d) Group comparisons (±s.e.m.) between amputees (amp) 2-handed intact controls (2H) and congenital 1-handed controls (1H) and correlations with phantom pain for: (b) activation during phantom/non-dominant hand movements (t(37)=−0.81,P=0.423;t(26)=−2.95,P=0.007;r(15)=0.67,P=0.003), (c) grey matter volume (t(38)=−2.92,P=0.006;t(27)=2.49,P=0.019;r(16)=0.60,P=0.009) and (d) functional connectivity between bilateral hand regions during rest in the phantom cortex (t(37)=−2.63,P=0.012;t(27)=−0.57,P=0.57;r(16)=−0.62,P=0.006). Means and s.e.’s of the two control groups are superimposed on thexaxis. Asterisks denote significance levels ofP<0.025. Preserved functional representation of the missing hand To assess changes in the primary sensorimotor hand area relating to phantom experiences, we studied 18 individuals with unilateral upper-limb amputation (amputees, Table 1 ), as well as 11 individuals with a congenital unilateral upper-limb deficiency and no phantom sensations (one-handers, Table 2 ), and 22 intact controls (two-handers), using magnetic resonance imaging (MRI). To functionally localize the cortical representation of the missing hand, participants underwent a functional MRI scan, while moving each hand separately (intact and phantom). One-handers were instructed to imagine moving their missing hand, as they did not have phantom limbs. Despite the long durations since amputation (18 years on average), significant activation was identified in the primary somatosensory cortex contralateral to the phantom hand in nearly all amputees ( Fig. 1a ). 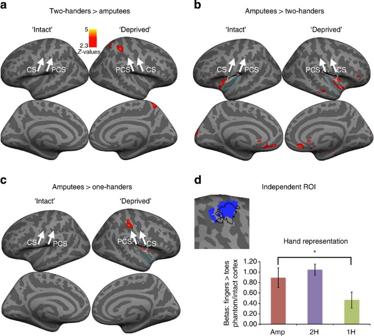Figure 3: Whole-brain group comparisons during non-dominant/missing-hand movements. Contrasts between the amputees and 2-handed controls (a,b) showed no differences in the primary sensorimotor cortex. Amputees showed increased activations in the posterior insula bilaterally. According to the Juelich atlas, peak voxels were located in the cytoarchitechtonic areas OP3 (white border) and Id1 (blue border). In addition, increased activation was shown in the orbitofrontal cortex bilateraly, as well as in medial occipital cortex of the intact hemisphere. A contrast with the 1-handed controls (c) showed increased activation in the primary sensorimotor cortex of amputees. This contrast also showed increased activation in the posterior insula contralateral to the missing hand (areas OP3 and Id1). To further confirm that the differences between phantom and imagined movements are not biased by the ROI used in the main test, a mirror ROI of the intact hand ROI (based on a conjunction of the three groups) was studied (see blue cluster in (d), with the borders of the original ROI superimposed in black). The beta values (±s.e.m) for the non-dominant/missing hand were significantly different compared with the 1-handed group (t(26)=−2.54,P=0.017), but not the 2-handed group (t(37)=−0.95,P=0.347). PCS, postcentral sulcus, CS, central sulcus, ‘Intact’ refers to the hemisphere contralateral to the intact/dominant hand cortex. ‘Deprived’ refers to the hemisphere contralateral to the phantom/non-dominant hand. Asterisks denote significance levels ofP<0.025. Indeed, group activation for phantom movements was similar to that found during two-handers’ non-dominant hand movements in the primary sensorimotor cortex ( Figs 2a and 3a , Table 3 ), suggesting preserved functional representations. Table 1 Amputee clinical details and imaging values in the phantom cortex. Full size table Table 2 1-Handed controls’ clinical details and imaging values in the contralateral sensorimotor cortex. Full size table Figure 1: Individuals’ missing-hand representations. Activation for movement of phantom hand versus toes in amputees ( a ) and for imagined missing-hand movements versus toes in 1-handed controls ( b ), projected on individuals’ inflated contralateral hemisphere. Arrows indicate the position of the central sulcus. Amputees are ordered according to their phantom pain ratings (amputees with greater chronic pain are presented first). Participants’ codes (A01, C01 and so on) correspond to Tables 1 and 2 . Full size image Figure 2: Chronic phantom pain relates to maintained local cortical representations and disrupted inter-regional connectivity. ( a ) Activation for movement of non-dominant and phantom hands versus toes in 2-handed controls (top) and amputees (bottom), projected on an inflated contralateral hemisphere. PCS, postcentral sulcus; CS, central sulcus. Black line delineates the boundaries of the ‘phantom cortex’ ROI. ( b – d ) Group comparisons (±s.e.m.) between amputees (amp) 2-handed intact controls (2H) and congenital 1-handed controls (1H) and correlations with phantom pain for: ( b ) activation during phantom/non-dominant hand movements ( t (37) =−0.81, P =0.423; t (26) =−2.95, P =0.007; r (15) =0.67, P =0.003), ( c ) grey matter volume ( t (38) =−2.92, P =0.006; t (27) =2.49, P =0.019; r (16) =0.60, P =0.009) and ( d ) functional connectivity between bilateral hand regions during rest in the phantom cortex ( t (37) =−2.63, P =0.012; t (27) =−0.57, P =0.57; r (16) =−0.62, P =0.006). Means and s.e.’s of the two control groups are superimposed on the x axis. Asterisks denote significance levels of P <0.025. Full size image Figure 3: Whole-brain group comparisons during non-dominant/missing-hand movements. Contrasts between the amputees and 2-handed controls ( a , b ) showed no differences in the primary sensorimotor cortex. Amputees showed increased activations in the posterior insula bilaterally. According to the Juelich atlas, peak voxels were located in the cytoarchitechtonic areas OP3 (white border) and Id1 (blue border). In addition, increased activation was shown in the orbitofrontal cortex bilateraly, as well as in medial occipital cortex of the intact hemisphere. A contrast with the 1-handed controls ( c ) showed increased activation in the primary sensorimotor cortex of amputees. This contrast also showed increased activation in the posterior insula contralateral to the missing hand (areas OP3 and Id1). To further confirm that the differences between phantom and imagined movements are not biased by the ROI used in the main test, a mirror ROI of the intact hand ROI (based on a conjunction of the three groups) was studied (see blue cluster in ( d ), with the borders of the original ROI superimposed in black). The beta values (±s.e.m) for the non-dominant/missing hand were significantly different compared with the 1-handed group ( t (26) =−2.54, P =0.017), but not the 2-handed group ( t (37) =−0.95, P =0.347). PCS, postcentral sulcus, CS, central sulcus, ‘Intact’ refers to the hemisphere contralateral to the intact/dominant hand cortex. ‘Deprived’ refers to the hemisphere contralateral to the phantom/non-dominant hand. Asterisks denote significance levels of P <0.025. Full size image Table 3 Functional location parameters for whole-brain contrasts between amputees and controls. Full size table This finding was further confirmed using a functional region of interest (ROI) analysis of the former hand area: activation during phantom movements did not differ significantly from activation during non-dominant hand movements of the two-handers group ( t (37) =−0.81, P =0.423; Fig. 2b ) or from intact hand movements in amputees’ ipsilateral hemisphere ( t (16) =−1.62, P =0.126). However, phantom activity was significantly greater than that seen in one-handers, who were instructed to imagine moving their missing hand ( t (26) =−2.95, P =0.007, Figs 1b , 2b and 3c ). To check whether the null results for the amputees could be due to insufficient statistical power, we considered the effect sizes for one-handers missing-hand movements (versus two-handers non-dominant hand: Cohen’s d =2.59; versus one-handers intact hand: Cohen’s d =2.49) and used these to perform post hoc power calculations, which confirmed that the subject numbers used here should comfortably detect such effects if present ( P <0.001). The preserved activity seen in amputees could potentially arise from associated movements of the residual arm, if the representation of the residual arm has expanded into the deprived hand cortex in the amputees. However, we found no evidence for increased representation of the residual arm of amputees in the phantom cortex (using an equivalent ratio to that used to assess phantom representation; t (37) =1.06, P =0.294). Functional correlates of phantom pain Next, we examined the relationship between phantom pain and movement-related functional MRI (fMRI) signal in the phantom hand area. According to the reorganizational model, maladaptive plasticity is expressed in shifted representation of the lips towards the former hand area, predicting increased activity within the phantom cortex during lip movements. To identify cortical representation of the lips, participants were asked to perform lip-smacking movements as a separate fMRI condition. We were unable to identify significantly increased activation during lip movements in amputees, compared with the 2-handed controls, in the phantom hand ROI ( t (37) =0.122, P =0.904). Furthermore, in the amputees group, the correlation between activation during lip movements and phantom pain magnitude was not significant ( r (15) =0.17, P =0.512). We then considered activation during phantom hand movement. Consistent with the persistent representation model, and contrary to the reorganization model, activation during phantom movements correlated with subjective ratings of chronic phantom pain magnitude in amputees ( r (15) =0.67, P =0.003): individuals with a worse history of phantom pain showed greater activation during phantom movements ( Fig. 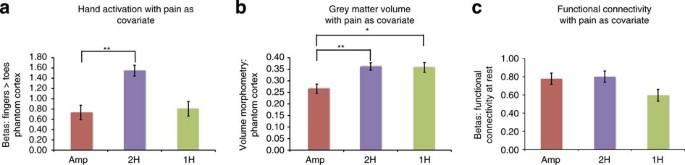Figure 4: Sensory loss in amputees relates to disrupted local cortical representations and preserved inter-regional connectivity. In order to expose the net effect of sensory loss in the amputee group, we statistically removed the effects of phantom pain magnitude from the group comparisons, using covariance analysis. Group comparisons (±s.e.m) between amputees (amp) 2-handed intact controls (2H) and congenital 1-handed controls for: (a) activation during phantom/non-dominant hand movements (F(1,36)=17.5,P=0.001;F(1,25)=0.09,P=0.769), (b) grey matter volume (F(1,37)=15.01,P=0.001;F(1,26)=8.34,P=0.008) and (c) functional connectivity between bilateral hand regions during rest in the phantom cortex (F(1,36)=0.09,P=0.768). This analysis revealed significant functional and structural disrupted representation in amputees, compared with the 2-handed controls. In contrast, differences between amputees and two-handers for functional connectivity at rest became nonsignificant following the pain covariance analysis. These results suggest that two complementary processes—phantom pain and sensory loss—modulate functional and anatomical representation in the phantom hand area. Asterisks denote significance levels of *P<0.025; **P<0.005. 2b and Table 4 ). This correlation was significantly stronger than that found between phantom pain and activation during lip movement ( Z =1.69, P =0.045). Furthermore, the correlation between habitual phantom pain and phantom activation remained significant while accounting for phantom pain rating on the day of the scan ( r (14) =0.62, P =0.011), suggesting that maintained representation is associated with chronic, rather than transient, phantom pain representation. Table 4 Pearson’s coefficients of determination ( r 2 ) between amputee clinical details and phantom cortex imaging values. Full size table As activation during phantom movements was greater in amputees suffering from worse phantom pain, does phantom pain contribute to the apparently maintained functional representation observed in the amputees’ group results (where no group differences were found between amputees and 2-handed controls)? We used covariate analysis to statistically remove the effects of phantom pain from the group comparisons, thereby ‘exposing’ other underlying effects. This procedure revealed a significant reduction in amputees’ phantom hand activation compared with 2-handed controls ( F (1,36) =17.5, P =0.001), but not compared with the one-handers ( F (1,25) =0.09, P =0.769, Fig. 4a ). This result demonstrates that at least two complementary processes—phantom pain and sensory deprivation—modulate functional representation in the phantom hand area in amputees: while loss of sensory input is associated with reduced functional representations, phantom pain experience is associated with increased representations. Figure 4: Sensory loss in amputees relates to disrupted local cortical representations and preserved inter-regional connectivity. In order to expose the net effect of sensory loss in the amputee group, we statistically removed the effects of phantom pain magnitude from the group comparisons, using covariance analysis. Group comparisons (±s.e.m) between amputees (amp) 2-handed intact controls (2H) and congenital 1-handed controls for: ( a ) activation during phantom/non-dominant hand movements ( F (1,36) =17.5, P =0.001; F (1,25) =0.09, P =0.769), ( b ) grey matter volume ( F (1,37) =15.01, P =0.001; F (1,26) =8.34, P =0.008) and ( c ) functional connectivity between bilateral hand regions during rest in the phantom cortex ( F (1,36) =0.09, P =0.768). This analysis revealed significant functional and structural disrupted representation in amputees, compared with the 2-handed controls. In contrast, differences between amputees and two-handers for functional connectivity at rest became nonsignificant following the pain covariance analysis. These results suggest that two complementary processes—phantom pain and sensory loss—modulate functional and anatomical representation in the phantom hand area. Asterisks denote significance levels of * P <0.025; ** P <0.005. Full size image Structural correlates of phantom pain We also examined changes in grey matter volume in the phantom hand area. Grey matter volume was significantly reduced in amputees’ phantom cortex, compared with two-handers corresponding hand cortex ( t (38) =−2.92, P =0.006; Fig. 2c ), as well as with the intact hand cortex in amputees ( t (17) =3.86, P =0.001), suggesting structural degeneration with loss of sensory inputs. However, we also found reduced grey matter volume in amputees’ phantom cortex compared with one-handers ( t (27) =2.49, P =0.019; Fig. 2c ), suggesting distinct processes for early versus late sensory deprivation. The reduction in grey matter volume in amputees compared with both control groups was little affected by covarying out the contribution of phantom pain ( F (1,37) =15.01, P =0.001; F (1,26) =8.34, P =0.008; Fig. 4b ). Within the amputee group, grey matter volume was modulated by chronic phantom pain: grey matter volume was greater in individuals with worse phantom pain ( r (16) =0.60, P =0.009, Fig. 2c , Table 4 ). Therefore, while acquired sensory loss seems generally to precipitate local structural degeneration in the deprived cortex, the experience of persistent phantom pain sensations, such as painful sensations triggered by peripheral inputs [8] , appears to maintain local structure, consistent with our fMRI results and the persistent representation model. Disrupted functional connectivity is linked with phantom pain Finally, given that phantom experiences are isolated from other sensory experiences, such as those typical of bimanual movements, we predicted that the phantom cortex would decouple from its contralateral counterpart (the intact hand area). We found that inter-hemispheric functional connectivity in amputees was significantly reduced compared with two-handers ( t (37) =−2.63, P =0.012), but did not differ significantly from one-handers ( t (27) =−0.57, P =0.57) ( Fig. 2d ). We also found that individuals suffering more from phantom pain showed greater reduction in inter-hemispheric functional connectivity ( r (16) =−0.62, P =0.006, Fig. 2d , Table 4 ). To tease apart the relative contribution of sensory loss from phantom pain, we applied the pain covariance analysis described above. After accounting for phantom pain, the group difference between amputees and two-handers became nonsignificant ( F (1,36) =0.09, P =0.768; Fig. 4c ), whereas a comparison with the one-handers group showed a trend towards increased connectivity in amputees ( F (1,26) =3.274, P =0.082). This suggests that, within the amputee group, persistent phantom pain representation may contribute to functional isolation of the phantom cortex from the sensorimotor system. Our results prompt a reassessment of the link between phantom pain and brain reorganization. While the maladaptive plasticity model suggests that greater pain should be associated with increased local reorganization, our results suggest instead that multiple factors interact to maintain local structural and functional representations but disturb long-range connectivity. We demonstrated comparable patterns of movement-related activity when amputees moved their phantom hand compared with 2-handed controls moving their non-dominant hand. This is in accordance with recent fMRI findings indicating maintained representation of the phantom hand in the primary sensorimotor cortex following amputation [6] , [9] , as well as no remapping in the visual cortex of individuals suffering from adult-onset visual deprivation [10] . We took advantage of this phenomenon to study patterns of structural and functional reorganization within the phantom cortex using a range of MRI modalities. People with acquired limb amputation and subsequent sensory deprivation, but not people with congenital limb absence, show structural degeneration of the phantom cortex. This result is in agreement with post-mortem histological observations in amputees [11] and recent neuroimaging findings [12] , [13] , associating loss of sensory input with neurodegeneration. Crucially, however, if amputees experience chronic phantom pain sensations, this is associated with preserved local functional and structural representations of the missing hand. A different picture is found when considering long-range interactions within the sensorimotor system: both acquired and congenital limb absence is associated with reduced inter-hemispheric functional connectivity, perhaps reflecting the longstanding lack of co-activation between the cortex representing the intact and absent limbs. This functional decoupling could be related to a recently documented decrease in callosal white-matter fractional anisotropy in lower-limb amputees [14] . Within the amputee group in the current study, phantom pain representation was found to further contribute to functional decoupling, as greater pain was associated with reduced connectivity. We therefore propose that cortical changes following limb amputation are most likely due to a combination of loss of sensory inputs and phantom pain experience. Sensory deprivation may result in disrupted functional and structural local cortical representations. On top of this background of reduced local representations, chronic phantom pain experience, such as triggered by bottom–up nociceptive inputs [8] or by top–down inputs from pain-related brain regions, maintains local cortical representations and disrupts inter-regional connectivity. We suggest that future accounts of cortical reorganization following sensory deprivation should consider both sensory loss and experience as potential drivers of plasticity. Participants Eighteen unilateral upper-limb amputees (mean age±s.e.m=46±3, six right-arm amputees), 22 age- and education-matched healthy controls (two-handers, age=41±3, seven with a dominant left hand), and 11 individuals with a congenital unilateral upper-limb deficit (one-handers, age=35±4, three missing the right hand) were recruited through the Oxford Centre for Enablement and Opcare in accordance with NHS National Research Ethics Service Approval (10/H0707/29), and written informed consent was obtained. Data from one amputee and one two-hander were discarded from the motor and functional connectivity analyses (respectively), owing to excessive head movements (>3 mm). Pain and phantom sensations ratings None of the 1-handed controls experienced phantom sensations ( Table 2 ). Amputees rated the frequencies of phantom/stump pain and non-painful phantom sensations, as experienced within the last year, as well as intensity of worst pain experienced during the last week (or in a typical week involving phantom/stump sensations). ‘Pain magnitude’ was calculated by dividing pain intensity (0: ‘no pain’—10: ‘worst pain imaginable’) by frequency (1—‘all the time’, 2 —‘daily’, 3—‘weekly’, 4—‘several times per month’ and 5—‘once or less per month’). This measure therefore reflects the chronic aspect of the pain as it combines both frequency and intensity, as used previously [15] . A similar measure was obtained for non-painful phantom vividness. Ratings of current pain/vividness were also obtained just before the scan. Scanning procedures Functional connectivity Participants were asked to lie still for 5 min in a dimmed room with their eyes open. Motor scan Participants were visually instructed to move either the left/right hand (finger movements), left/right arm (elbow movements), feet (bilateral toe movements) or lips. Participants who did not experience vivid phantom sensations (two amputees and all 1-handed controls) were instructed to imagine moving their missing hand (if elbow intact) and arm (if elbow absent). The protocol comprised of alternating 12 s periods of movement and ‘rest’. Each of the six conditions was repeated four times, in a counterbalanced manner. Participants received extensive training on the degree and form of movements expected, including phantom movements. It was stated clearly that amputees with phantom sensation were required to perform actual movements with their phantoms, rather than motor imagery. The amputees were asked to demonstrate to the experimenter the degree of volitional movement in the phantom using their intact hand. When in doubt, stump muscles were palpated by the experimenter to verify that actual movements were executed during movement of the phantom. In the scanner, correct task performance was verified visually both on- and offline using video recordings. To confirm that movements were made at the instructed times, phantom movements execution was verified in a subset of five amputees using electromyography recordings from arm muscles during the scan. MRI data acquisition The MRI measurements were obtained using a 3-Tesla Verio scanner (Siemens, Erlangen, Germany) with a 32-channel head coil. Anatomical data were acquired using a T1-weighted magnetization prepared rapid acquisition gradient echo sequence with the parameters: TR=2040, ms; TE=4.7 ms; flip angle=8° and voxel size=1 mm isotropic resolution. Functional data based on the blood oxygenation level-dependent signal were acquired using a multiple gradient echo-planar T2*-weighted pulse sequence, with the parameters: TR=2000, ms, TE=30 ms, flip angle=90°, imaging matrix=64 × 64 and FOV=192 mm axial slices. Forty-six slices with slice thickness of 3 mm and no gap were oriented in the oblique axial plane, covering the whole cortex, with partial coverage of the cerebellum. Preprocessing and statistical analysis All imaging data were processed using FSL 5.1 ( www.fmrib.ox.ac.uk/fsl ). Data collected for individuals with absent right hands were mirror reversed across the mid-sagittal plane before all analyses so that the ‘deprived’ hemisphere was consistently aligned. Data collected for an equal proportion of left-hand-dominant two-handers was also flipped, in order to account for potential biases stemming from this procedure. Functional analysis Functional data were analysed using FMRIB’s expert analysis tool (FEAT, version 5.98). The following pre-statistics processing was applied to each individual run: motion correction using FMRIB’s Linear Image Registration Tool (MCFLIRT [16] ); brain extraction using BET [17] ; mean-based intensity normalization; spatial smoothing using a Gaussian kernel of FWHM (full width at half maximum) 5 or 6 mm (for task-based and resting scans, respectively); and highpass temporal filtering of 300 and 150 s (respectively). Time-series statistical analysis was carried out using FILM (FMRIB’s Improved Linear Model) with local autocorrelation correction. Functional data were aligned to structural images (within-subject) initially using linear registration (FMRIB’s Linear Image Registration Tool, FLIRT), then optimized using Boundary-Based Registration [18] . Structural images were transformed to standard MNI space using a nonlinear registration tool (FNIRT), and the resulting warp fields applied to the functional statistical summary images. To compute parameter estimates, we applied a voxel-based general linear model (GLM), as implemented in FEAT. For the task-based scans, the block design paradigm was convolved with a gamma function [19] , and its temporal derivative was used to model the activation time course. Three main contrasts were defined between different task movement types: (i) intact (or dominant) hand versus feet; (ii) affected (or non-dominant) hand versus feet; and (iii) lips versus feet. Individual maps for contrast (ii) are presented in Fig. 1 . For presentation purposes, the activation maps were smoothed using a FWHM of 2.5 mm, and thresholds were adjusted using a false discovery rate of P <0.05 (with the exception of amputees A06, A10 and A16, and one-handers C1, C6 and C11, which were threholded at Z >2). For resting state scans, individual time series from the intact/dominant cortex were extracted using a group ROI (see below) and used as individual ‘seeds’ to model the activation time course for a further first-level FEAT analysis (with white matter and cerebrospinal fluid time series as nuisance regressors). Head motion parameters were included as nuisance regressors in individual scans. For presentation purposes, individual, statistical parametric activation maps with the first contrast were projected on individuals’ inflated brains, using FreeSurfer ( http://surfer.nmr.mgh.harvard.edu/ ). Group level analysis was carried out using FMRIB’s Local Analysis of Mixed Effects [20] . The cross-subject GLM included the three groups. Z (Gaussianised T/F) statistic images were thresholded using clusters determined by Z >2 and a family-wise-error-corrected cluster significance threshold of P <0.05 was applied to the suprathreshold clusters. To functionally define hand ROIs, inter-group means were calculated from the motor scans using the following conjunctions: (i) intact/dominant hand movements in all three groups, using a threshold of Z >8; (ii) phantom/non-dominant hand movements in amputees and two-handers, using a threshold of Z >7. These thresholds yielded clusters comparable in size, centred around the hand knob of the central sulcus used for the ROI analysis. In addition, the intact cortex ROI was mirror reversed across the mid-sagittal plane and used as an independent ROI ( Fig. 3d ). Whole-brain differences between the amputees group and each of the control groups (two-handers and one-handers) were tested for non-dominant/phantom/missing-hand movements. In addition, a contrast between elbow and feet movements was tested at both levels, to determine whether remapping of elbow representations contributed to our results. For presentation purposes, statistical parametric activation maps were projected on the inflated surface of a representative participants’ cortex or a standard MNI brain, using Freesurfer. Structural analysis Whole-brain analysis was carried out using a voxel-based morphometry-style analysis (FSL-VBM) [21] using default settings as described at www.fmrib.ox.ac.uk/fsl/fslvbm/ . In brief, brain extraction and tissue-type segmentation were performed and resulting grey matter partial volume images were aligned to standard space using first linear (FLIRT) and then nonlinear (FNIRT) registration tools. The resulting images were averaged, modulated and smoothed with an isotropic Gaussian kernel of 3 mm FWHM to create a study-specific template, based on 11 participants from each of the three groups, and the grey matter images of all participants were re-registered to this, including modulation by the warp field Jacobian. ROI analysis For group comparisons, individual values for VBM and GLM parameter estimates (betas) from the low-level motor scan (converted to percentage signal change) were extracted for each of the hand ROIs. Individual values from the ‘phantom’ ROI were divided by the corresponding values from the ‘intact’ ROI, and used for group comparisons. Betas from the functional connectivity study were extracted from the phantom hand area. The values extracted from the phantom hand ROI were used for correlation analyses. Statistical analysis Statistical analysis was carried out using SPSS version 18. Data sets were initially assessed for normality, using the Shapiro–Wilk test. Within group, means were statistically compared using paired two-tailed student t -tests. Between-group effects were initially statistically compared using one-way analysis of variance. As all analysis of variance tests were found significant (Motor scan: F (2,47) =7.21, P =0.002; grey matter volume: F (2,48) =4.28, P =0.019; Functional connectivity: F (2,47) =4.45, P =0.017), the means of the amputees group were further compared with each of the control groups (two-handers and one-handers), using independent samples two-tailed t -tests. The level of significance for group comparisons was therefore adjusted to the value P <0.025 to account for multiple comparisons. Where significant departure from normality was found, the t -test results were further verified using non-parametric tests (Mann–Whitney or Wilcoxon, as appropriate). To account for potential confounds of unbalanced statistical design, the independent-sample t -tests reported in Fig. 2 were further tested using a Mann–Whitney test, which confirmed the significance of the reported results, at the level P <0.005, with the exception of the comparison between amputees and one-handers grey matter volume ( P =0.16). A separate covariate of phantom pain was used in order to identify deprivation-related group differences. Correlations were evaluated using a two-tailed Pearson’s correlation coefficient, and were further tested using a ( n −1) jackknife approach. Comparisons between correlations was performed using Fisher’s r to Z transformation. Power calculations were performed based on the effect size shown between one-handers and two-handers during non-dominant/missing-hand movements (Cohen’s d =2.59 and 2.49 for between- and within-group comparisons). Covariates To rule out that interactions between the three imaging measurements were driving the reported correlations with chronic phantom pain, and to better characterize the chronic aspect of phantom pain, we calculated each of the original correlations while taking into account the partial contributions of the two other variables, and of transient phantom pain ratings (as taken before the scan). The resulting correlation with chronic phantom pain were r (15) =0.51, P =0.064 (phantom representation), r (16) =0.55, P =0.040 (grey matter volume) and r (16) =−0.58, P =0.030 (functional connectivity). How to cite this article: Makin, T. R. et al . Phantom pain is associated with preserved structure and function in the former hand area. Nat. Commun. 4:1570 doi: 10.1038/ncomms2571 (2013).